3D niche microarrays for systems-level analyses of cell fate The behaviour of mammalian cells in a tissue is governed by the three-dimensional (3D) microenvironment and involves a dynamic interplay between biochemical and mechanical signals provided by the extracellular matrix (ECM), cell–cell interactions and soluble factors. The complexity of the microenvironment and the context-dependent cell responses that arise from these interactions have posed a major challenge to understanding the underlying regulatory mechanisms. Here we develop an experimental paradigm to dissect the role of various interacting factors by simultaneously synthesizing more than 1,000 unique microenvironments with robotic nanolitre liquid-dispensing technology and by probing their effects on cell fate. Using this novel 3D microarray platform, we assess the combined effects of matrix elasticity, proteolytic degradability and three distinct classes of signalling proteins on mouse embryonic stem cells, unveiling a comprehensive map of interactions involved in regulating self-renewal. This approach is broadly applicable to gain a systems-level understanding of multifactorial 3D cell–matrix interactions. Over the last decades, three-dimensional (3D) cell culture matrices extracted from natural extracellular matrix (ECM), such as collagen or Matrigel TM , have been extensively applied as model systems to elucidate complex cell behaviour [1] , [2] , notably in the fields of cancer or stem cell research. It has been shown that these environments, in contrast to two-dimensional (2D) cell culture systems, allow for gene expression patterns and cellular phenotypes that often more closely resemble those found in vivo [3] , [4] . However, these naturally derived 3D culture systems suffer from relatively poorly defined compositions and batch-to-batch variation. For many fundamental biological studies, they also lack the flexibility of altering their properties in systematic ways. For example, biophysical properties such as stiffness or porosity are tightly linked to the signalling properties of a 3D matrix, making an independent control of the key matrix parameters nearly impossible. Hence, with one formulation of such a matrix at hand, it is impossible to gain an in-depth understanding of the individual signals and their coordinated action on cell fate in 3D. The recent use of spotting robots to microarray polymeric cell culture substrates with modular physical properties such as surface roughness and wettability [5] , as well as combinatorial mixtures of ECM proteins and recombinant growth factors [6] , [7] , [8] , have provided paths forward in dissecting the complexity of extrinsic cell fate regulation in vitro . However, these approaches have all been limited to 2D and it has, thus far, not been possible to reconstruct physiologically relevant 3D in vitro microenvironments to test such multiple biochemical and mechanical cues in a systematic way. In this work, we have developed an experimental paradigm which demonstrates for the first time the necessary flexibility and throughput to rapidly and efficiently modulate the interaction between the various components of the cellular microenvironment in 3D space, and to interrogate cell behaviour at scales down to single-cell resolution. This approach, based on a combination of biomaterials engineering, liquid handling automation, multimodal readouts including high-throughput microscopy and flow cytometry, as well as customized bioinformatics tools, allows the discrete combinatorial modulation of the 3D cell microenvironment in highly parallelized manner. We illustrate here the power of this approach by deploying it to elucidate mechanisms controlling colony formation and self-renewal of single mouse embryonic stem cells (mESC), a model system with wide relevance for basic cell biology and regenerative medicine, for which precise understanding and control of cell fate is critical, and whose characteristic behaviour in 3D has remained largely unexplored. To realize a 3D screening of cellular microenvironments, it is necessary to engineer a biomaterials system composed of a library of molecular building blocks, which can be independently mixed and then cross-linked in the presence of cells to form a wide diversity of 3D cell environments with distinct and independently controllable mechanical and biochemical properties. To this end, we build on one of the approaches to engineer synthetic hydrogels as biomimetic 3D cell microenvironments with very well-defined physicochemical and biochemical properties [9] . We employ the coagulation enzyme-activated transglutaminase factor XIIIa (FXIIIa) to cross-link branched poly(ethylene glycol)-(PEG)-based macromers into 3D hydrogel networks ( Fig. 1a ) [10] . The derivatization of the PEG macromers with short peptidic substrates for FXIIIa allows site-specific enzymatically mediated amide bond formation between the PEG chain termini under physiological conditions. Indeed, single mESC encapsulated within these PEG-based hydrogels show a very good viability (89.1±7.3% s.d.) that is not significantly different ( P =0.44, two-sample unpaired t -test, unequal variance, two-tailed distribution) from standard culture conditions on gelatin-coated plastic (92.5±3.6% s.d.) ( Supplementary Fig. 1a ). Gel-encapsulated single cells are physically separated from each other from the beginning of an experiment and, in the case of an epithelial cell growth pattern, remain so over time, thereby expanding as clonal entities. 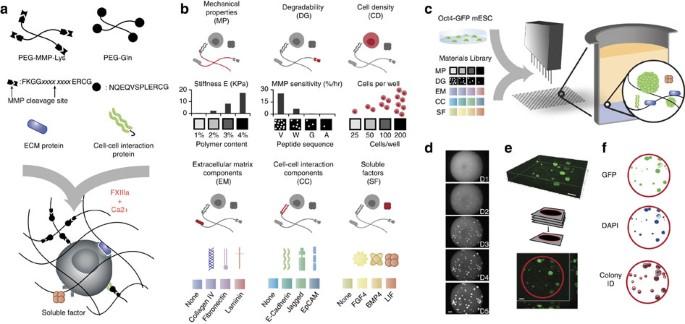Figure 1: 3D combinatorial screening from a modular materials library. (a) Enzymatically mediated cross-linking scheme, wherexxxx xxxxrepresents specific peptide sequence. (b) Components of the combinatorial toolbox are assembled from biologically relevant factors in categorized form. Stiffness and MMP sensitivity of the matrix are set within the experimentally measured ranges shown (n=3 replicates). (c) Experimental process consists of combining the components library with reporter cells using robotic mixing and dispensing technology into 1,536-well plates (n=3 replicates). (d–f) Automated microscopy and image processing to determine colony size and GFP intensity. Average cell density per well is set by the initial cell concentration used in the experiment, and exact initial cell density for each well is determined retrospectively by imaging. Examples of a set of images tracking colony growth in a single well over the course of a 5-day experiment (d) 3D confocal reconstruction (e) and image segmentation are shown (f). Scale bar, 200 μm. Figure 1: 3D combinatorial screening from a modular materials library. ( a ) Enzymatically mediated cross-linking scheme, where xxxx xxxx represents specific peptide sequence. ( b ) Components of the combinatorial toolbox are assembled from biologically relevant factors in categorized form. Stiffness and MMP sensitivity of the matrix are set within the experimentally measured ranges shown ( n =3 replicates). ( c ) Experimental process consists of combining the components library with reporter cells using robotic mixing and dispensing technology into 1,536-well plates ( n =3 replicates). ( d – f ) Automated microscopy and image processing to determine colony size and GFP intensity. Average cell density per well is set by the initial cell concentration used in the experiment, and exact initial cell density for each well is determined retrospectively by imaging. Examples of a set of images tracking colony growth in a single well over the course of a 5-day experiment ( d ) 3D confocal reconstruction ( e ) and image segmentation are shown ( f ). Scale bar, 200 μm. Full size image To allow for efficient growth in 3D, the gels can be rendered susceptible to cell-secreted proteolytic remodelling by designing PEG–peptide conjugates bearing an additional protease substrate site for gel degradation [11] , [12] ( Fig. 1a ). Moreover, biologically active molecules such as oligopeptides or proteins can be site-specifically tethered to the gel networks during the enzymatic gel cross-linking in the same reaction mixture ( Fig. 1a and Supplementary Fig. 1b,c ). Thus, we reasoned that this molecular tool kit for making hydrogel matrices should permit to probe a very large combinatorial space of different 3D cellular microenvironments. To establish this system and demonstrate its versatility, five key signal types of the 3D in vivo microenvironment were represented where each of these characteristics could be independently varied ( Fig. 1b ): matrix mechanical properties (abbreviated with ‘MP’), proteolytic degradability (‘DG’), extracellular matrix (‘EC’) proteins, cell–cell interaction (‘CC’) proteins and soluble factors (‘SF’). The Young’s moduli (E) of the gels were specified between ca . 300 and 5,400 Pa by varying the polymer content ( Fig. 1b and Supplementary Fig. 2 ) [13] . The gels were rendered differentially degradable by matrix metalloproteinases (MMPs) via the incorporation of peptides of different sensitivities ( k cat / K m ) to cell-secreted MMPs ( Supplementary Fig. 3 ) [12] . Importantly, we adjusted the precursor content of gels having different susceptibilities to MMP-mediated degradation in order to perfectly match their mechanical properties ( Supplementary Fig. 2 ). Thus, we could independently control key mechanical and biochemical properties of this synthetic gel system. To systematically modulate the cell signalling properties of the matrices, we chose a set of ECM and recombinant growth factor proteins, which had previously been implicated in regulating ESC pluripotency, and which we enzymatically tethered to the gels ( Fig. 1b and Supplementary Fig. 1b,c ). Indeed, ESC interaction with laminin, fibronectin and collagen IV had previously been associated with a loss of pluripotency in 2D [14] , however, ligation of their integrin homodimers by peptide analogues in a 3D culture system indicated that they could instead promote maintenance of self-renewal [15] . In addition, an increasing body of work has pointed to transmembrane proteins involved in cell–cell signalling as mediators of self-renewal: E-Cadherin, EpCam and the Notch ligand Jagged 1 have been chosen here as representative examples [16] , [17] , [18] , [19] . Finally, we added the soluble ESC regulatory factors leukemia inhibitory factor (LIF), bone morphogenetic protein 4 (BMP4) and fibroblast growth factor 4 (FGF4) [14] , [20] to a serum-free medium formulation such that they could reach the encapsulated cells via the diffusive properties of the gel network. In our current experimental scheme, we specify four levels of modulation for each of the five categories, leading to a total parameter space of 1,024 unique conditions ( Fig. 1c and Supplementary Fig. 4 ). In addition, cell density, increasingly recognized as an important modulator of ESC fate by autocrine effects, could be prescribed in this experimental setup as well as retrospectively imaged. This level of complexity in formulating 3D cell-containing gels, as well as the required repetitions, can only be reduced to practice by miniaturizing the sample volumes and adapting automated methods for gel synthesis ( Fig. 1c ) and cell fate analysis ( Fig. 1d–f ). We use a programmable nanolitre-range liquid handling robot equipped with small-volume dispensing tips to accurately synthesize 1 μl of each of the unique conditions in triplicate, in a completely automated manner, onto glass slides (not shown) or into standard 1,536-well plates ( Supplementary Fig. 4 ). The latter format was chosen as it presented an ideal surface-to-volume ratio for our selected hydrogel drops and represented a standard format that could be adapted to various experimental setups and adopted by others with access to this type of instrumentation. Furthermore, by physically isolating each well from its neighbours (in contrast to the slide format), we could consider each condition as a truly independent experimental condition free of cross-contamination. Once the 3D gel array is generated, the system can function as a truly multimodal assay platform, where multiple readouts can be obtained in parallel. To obtain quantitative information on ESC self-renewal and differentiation in response to the above 3D microenvironment array, we made use of an Oct4-GFP reporter cell line, in conjunction with automated imaging and image analysis ( Fig. 1e,f ). The transcription factor Oct4 is widely considered as a marker of embryonic stem cell pluripotency [21] . Cells embedded in PEG hydrogels were imaged the day following seeding to obtain the actual initial number of cells for each well. In the most permissive conditions, these cells formed spherical colonies within 3 days and kept proliferating until fixation 5 days after gel embedding ( Fig. 1d ). High-resolution confocal microscopy confirmed that colonies growing in these conditions were in a 3D space of ~500 μm in thickness ( Fig. 1e ), and that soluble molecules in the medium could rapidly diffuse homogeneously throughout the thickness of the gel ( Supplementary Fig. 5 ). Automated imaging was performed at a low magnification to capture an entire well in a field of view. Using a low numerical aperture objective also allowed us to capture the complete 3D architecture of the hydrogel at the bottom of the well with a relatively low number of z -stacks. To correctly segment colonies, we developed an automated analysis procedure. Although a large number of morphometric readouts could be obtained from these images, we focused here on colony area as a measure of proliferation, and GFP intensity as a measure of ESC pluripotency ( Fig. 1f ). For every unique combination of MP, DG, EC, CC and SF, colony area and GFP intensity were calculated as the average of three replicates, and organized by input condition ( Fig. 2a ). Notably, soluble factor modulation was found to be the strongest predictor of heat map intensity, with the LIF condition clearly leading to both high proliferation and self-renewal, with the opposite effect for FGF4 and BMP4, and an intermediate regime appearing for conditions with no soluble factors. The top ten self-renewing and proliferating conditions were all within the LIF condition, and most tended to be in conditions of low mechanical properties and absence of cell–cell interaction proteins. Indeed, when all microenvironments were plotted as colony area versus GFP intensity ( Fig. 2b ), three clusters emerged that were identified as the LIF, no factors (‘None’) and BMP4/FGF4 populations, with very little overlap between them. The LIF dependence proved to be a strong biological validation of the platform, as LIF is known to be a potent mediator of ESC self-renewal via phosphorylation of the transcription factor STAT3 (signal transducer and activator of transcription 3). In addition, distinct area versus GFP relationships emerged out of such a representation, suggesting that the correlation between self-renewal and proliferation is linked to a particular soluble factor regime; for FGF/BMP, irrespective of growth characteristics, self-renewal was lost, whereas with LIF proliferation was strongly correlated to self-renewal. In microenvironments devoid of any exogenous soluble factors, the existence of self-renewing colonies pointed to the potential role of other factors involved in maintaining ESC in 3D. Interestingly, the most self-renewing and proliferating (i.e., high GFP and high area) matrix characteristics in all subpopulations were found in conditions of low matrix stiffness ( Fig. 2c,d ). 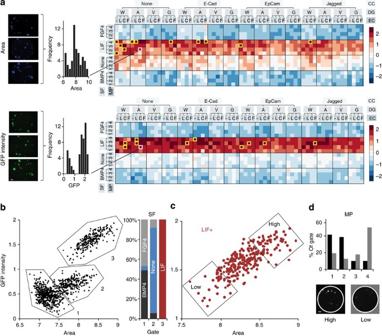Figure 2: ESC proliferation and self-renewal by input conditions. (a) Image analysis is carried out for each well in DAPI and GFP channels, triplicates of each unique experimental condition are analysed and represented as heat maps. Data is log-transformed, normalized and centred about the mean. Yellow boxes denote top 10 conditions out of the 1,024 unique conditions. (V, W, G, A: degradabilities in decreasing order of MMP sensitivity; –, L, C, F: none, laminin, collagen IV, fibronectin; 1, 2, 3, 4: mechanical properties categories, in increasing stiffness). (b) Gating of all unique conditions and identification of soluble factor composition within these gates. (c) Selection of LIF(+) population, gating for high- and low-area GFP populations and (d) analysis of mechanical properties distribution within these two populations. Scale bar, 200 μm. Figure 2: ESC proliferation and self-renewal by input conditions. ( a ) Image analysis is carried out for each well in DAPI and GFP channels, triplicates of each unique experimental condition are analysed and represented as heat maps. Data is log-transformed, normalized and centred about the mean. Yellow boxes denote top 10 conditions out of the 1,024 unique conditions. (V, W, G, A: degradabilities in decreasing order of MMP sensitivity; –, L, C, F: none, laminin, collagen IV, fibronectin; 1, 2, 3, 4: mechanical properties categories, in increasing stiffness). ( b ) Gating of all unique conditions and identification of soluble factor composition within these gates. ( c ) Selection of LIF(+) population, gating for high- and low-area GFP populations and ( d ) analysis of mechanical properties distribution within these two populations. Scale bar, 200 μm. Full size image To quantify in a systematic way how self-renewal and proliferation varied as a function of the various microenvironments, we used generalized linear models (GLMs), which encompassed all of the five determinants of the microenvironment and their interactions (see model building in Methods) ( Fig. 3 ). This approach allowed us to explain more than 70% of the variability in the system. By decoupling subtle effects from the more dominant ones, we were able to uncover and quantify the relative importance of various factors ( Fig. 3a ), establishing a global hierarchy of components affecting ESC fate in 3D. Soluble factors accounted for >60% of the model variance. Physical properties, including matrix degradability and stiffness, accounted for approximately half of the remaining model variance, and tethered protein and initial cell density effects each accounted for at most 15%. We also investigated the role of individual factors within these categories ( Fig. 3b ). BMP4 and FGF4, when presented as single factors in serum-free medium as in this study, impaired self-renewal and no other microenvironmental factor could overcome this effect to any significant degree. Degradable matrices favoured self-renewal, but not necessarily proliferation. Thus, the physical parameters of the matrix may not only dictate colony growth but also coordinate stemness. These processes do not always act in parallel and may be mediated by interacting factors. Indeed, ECM proteins tended to increase the size of colonies but decreased Oct4 expression, which matched previous findings in 2D, where laminin and fibronectin were shown to enhance differentiation of ESC [14] . Surprisingly, cell–cell interaction proteins, such as EpCam, tended to decrease both proliferation and self-renewal in our system, although all three chosen proteins had been previously implicated in maintenance of ESC self-renewal in 2D studies [16] , [17] , [18] . This suggests that certain pathways could be differentially activated or overridden by alternative factors in a 3D environment [16] . 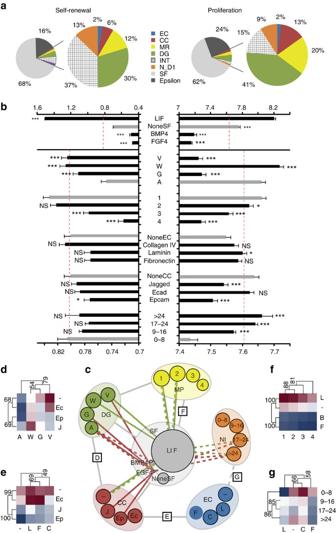Figure 3: Systems-level analyses at multiple scaling levels. (a) Role of factor categories and (b) of individual factors within categories in overall response. Grey bars represent baseline or control condition and dashed red line represents overall mean. (c) Network interaction map for significantly interacting categories. Grey lines indicate interactions shared by both area and GFP intensity, while green lines represents interactions present only for GFP intensity. Interactions having the most (green) and least (red) effect on proliferation (solid line) and self-renewal (dashed line) are indicated (top and bottom five interacting partners per category). (d–g) Examples of all pairwise interactions between two categories are shown as clustered heat maps, with minimum and maximum values within each heat map defining the colour range. (d–f) Interactions for area and (g) GFP intensity. Numbers along cluster branches indicate support level. Error bars represent s.e.m. V, W, G, A: degradabilities in decreasing order of MMP sensitivity; –, L, C, F: none, laminin, collagen, fibronectin; 1, 2, 3, 4: mechanical properties categories, in increasing stiffness; NI: number of cells per well at Day 1. Error bars represent s.e.m. All pairwise differences were computed using the Tukey–Kramer method. ***P<0.001, **P<0.01, *P<0.05. Figure 3: Systems-level analyses at multiple scaling levels. ( a ) Role of factor categories and ( b ) of individual factors within categories in overall response. Grey bars represent baseline or control condition and dashed red line represents overall mean. ( c ) Network interaction map for significantly interacting categories. Grey lines indicate interactions shared by both area and GFP intensity, while green lines represents interactions present only for GFP intensity. Interactions having the most (green) and least (red) effect on proliferation (solid line) and self-renewal (dashed line) are indicated (top and bottom five interacting partners per category). ( d – g ) Examples of all pairwise interactions between two categories are shown as clustered heat maps, with minimum and maximum values within each heat map defining the colour range. ( d – f ) Interactions for area and ( g ) GFP intensity. Numbers along cluster branches indicate support level. Error bars represent s.e.m. V, W, G, A: degradabilities in decreasing order of MMP sensitivity; –, L, C, F: none, laminin, collagen, fibronectin; 1, 2, 3, 4: mechanical properties categories, in increasing stiffness; NI: number of cells per well at Day 1. Error bars represent s.e.m. All pairwise differences were computed using the Tukey–Kramer method. *** P <0.001, ** P <0.01, * P <0.05. Full size image Synergistic or antagonistic effects between factors that were statistically significant were represented by a network interaction map ( Fig. 3c ) and as clustered heat maps showing significant pair-wise interactions ( Fig. 3d–g ). Although some interactions such as those involving soluble factors were involved both in self-renewal and proliferation, others were self-renewal specific ( Fig. 3c and Supplementary Fig. 6 ). For example, the presence of EpCam with all ECM proteins tended to reduce colony growth ( Fig. 3e ), while the presence of collagen in gels with low cell density tended to enhance self-renewal ( Fig. 3g ). Thus, ECM proteins, with their role in activating cell adhesion complexes via integrin engagement [15] , are involved in modulating the purely physical components of the matrix. Overall, the interaction scheme centred around the soluble factors, underscoring their key role in regulating ESC fate even in a 3D environment ( Fig. 3c ). Indeed, LIF potentiated the strongest synergistic effects on proliferation in degradable matrices, while its effect on self-renewal was most enhanced at high cell densities. It can be noted that LIF provided synergistic effects at low mechanical properties for both proliferation and self-renewal, emphasizing the key role of optimal stiffness in a 3D context. Conversely, the antagonistic effects of soluble factors on self-renewal were most significant at high cell densities and in non-degradable matrices, while for proliferation Epcam and Jagged were also involved. To study key aspects of ESC regulation in 3D uncovered by this large-scale screen in more detail, we rendered our platform compatible with complementary downstream cell assays including flow cytometry and quantitative reverse transcription PCR (RT–PCR) ( Fig. 4 ). These novel readouts were implemented in more targeted experiments ( Fig. 4a ) and in a time-lapse mode ( Fig. 4b ) to also uncover the dynamics of 3D ESC behaviour. For instance, we simultaneously investigated the potency of LIF by performing a dose-dependence study, evaluated the effect of mechanical properties by widening our stiffness range and retrospectively measuring the stiffness of every gel ( Supplementary Fig. 7 ), and explored a wider range of pre-set cell densities ( Fig. 4a ). 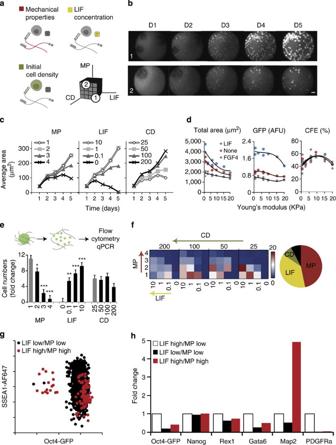Figure 4: Downstream cell assays are compatible with 3D gel microarray approach. (a) In a targeted screen, 4 levels of 3 factors are combined for a total of 64 unique conditions with multiple replicates. Mechanical properties are varied from 200 to 2,000 Pa (Young’s modulus E), LIF concentration varied from 103to 10 U ml−1(with negative control 0 U ml−1) and cell density varied from 25 to 200 cells per μl. (b) Images are taken every day, allowing for the observation of the evolution of colony growth over time in all conditions—here two selected conditions are shown: both start with an initial cell density of 200 cellsper μl; for condition 1: LIF=103U ml−1, MP=200 Pa (soft); for condition 2: LIF=10 U ml−1, MP=2,000 Pa (stiff). (c) After image analysis, measures such as average colony area can be assessed over time. (d) Average colony area, GFP intensity and colony-forming efficiency are shown as a function of the measured stiffness for three soluble factor regimes. (e) Dissociation of the hydrogel matrices in each well allows a quantification and phenotyping of cells by flow cytometry and other downstream assays. (f) Heatmap representation indicating a clear trend towards a graded bidirectional influence of LIF and MP, an observation reinforced by the global analysis. (g) Differences between specific conditions of interest can be further investigated by analysis of surface marker expression or (h) PCR analysis of genes involved in self-renewal and differentiation into early germ layer. Fold change here is with respect to the baseline LIF high/MP low condition (n=3 biological replicates). Scale bar, 200 μm. Error bars represent s.e.m. All pairwise differences were computed using the Tukey–Kramer method. ***P<0.001, **P<0.01, *P<0.05. Figure 4: Downstream cell assays are compatible with 3D gel microarray approach. ( a ) In a targeted screen, 4 levels of 3 factors are combined for a total of 64 unique conditions with multiple replicates. Mechanical properties are varied from 200 to 2,000 Pa (Young’s modulus E), LIF concentration varied from 10 3 to 10 U ml −1 (with negative control 0 U ml −1 ) and cell density varied from 25 to 200 cells per μl. ( b ) Images are taken every day, allowing for the observation of the evolution of colony growth over time in all conditions—here two selected conditions are shown: both start with an initial cell density of 200 cellsper μl; for condition 1: LIF=10 3 U ml −1 , MP=200 Pa (soft); for condition 2: LIF=10 U ml −1 , MP=2,000 Pa (stiff). ( c ) After image analysis, measures such as average colony area can be assessed over time. ( d ) Average colony area, GFP intensity and colony-forming efficiency are shown as a function of the measured stiffness for three soluble factor regimes. ( e ) Dissociation of the hydrogel matrices in each well allows a quantification and phenotyping of cells by flow cytometry and other downstream assays. ( f ) Heatmap representation indicating a clear trend towards a graded bidirectional influence of LIF and MP, an observation reinforced by the global analysis. ( g ) Differences between specific conditions of interest can be further investigated by analysis of surface marker expression or ( h ) PCR analysis of genes involved in self-renewal and differentiation into early germ layer. Fold change here is with respect to the baseline LIF high/MP low condition ( n =3 biological replicates). Scale bar, 200 μm. Error bars represent s.e.m. All pairwise differences were computed using the Tukey–Kramer method. *** P <0.001, ** P <0.01, * P <0.05. Full size image Proliferation was maintained in all conditions for the first 2 days, followed by a strong dependence on all three tested parameters ( Fig. 4c ). Notably, LIF maintained its proliferative role in 3D even at a concentration three orders of magnitude less than standard. We confirmed that proliferation was directly related to lower matrix stiffness, while an intermediate stiffness was found to be optimal for self-renewal and colony-forming efficiency ( Fig. 4d ). This finding is in line with data suggesting that 3D solid stress can control cellular growth at both the macroscopic and cellular levels in multicellular aggregates such as tumour spheroids [22] . More recent work has shown that the elasticity of the in vitro substrate can direct stem cell fate [23] , [24] . Our results suggest that mechanical properties could play a similar and fundamental role in regulating ESC maintenance in 3D, where optimal properties in the range of those measured in the early blastocyst might be most appropriate [25] , [26] . Hydrogel stiffness may indeed be mechanistically translated into such effects via YAP/TAZ activation, as has been shown in 2D [27] . To corroborate our findings at the colony level with single-cell flow cytometry data and gene expression information, we first developed a robotic process to dissociate the hydrogel matrix within each well with protease solution while maintaining cellular integrity. Total cell counts by flow cytometry were most closely correlated to a measure of total colony area by imaging ( Supplementary Fig. 8 ). To better define the role of cell density, we normalized total colony area by initial cell density: although higher initial cell densities led to larger colonies, this was not reflected in actual cell numbers counted by flow cytometry ( Fig. 4e ), suggesting that cells within larger colonies may have died. As with image-based data, each condition could be visualized individually; a heatmap representation ( Fig. 4f ) indicates a clear trend towards a graded bidirectional influence of LIF and MP, an observation reinforced by a global analysis showing the near-equal role of these two factors in influencing cell proliferation and the reduced role of cell density. An additional advantage of dissociating cells from the gels is the possibility to readily perform immunocytochemisty. Staining for SSEA1, a surface marker commonly used as a complementary marker of pluripotency to transcription factors such as Oct4, indicated a wide range of SSEA1 expression even in cases of high Oct4 ( Fig. 4g ); SSEA1 expression generally reached higher levels in softer matrices, and a SSEA1 high/Oct4 low subpopulation emerged in cases of high LIF and high MP, suggesting that some cells have acquired subtle modulations in intracellular and extracellular markers of pluripotency and may have initiated early differentiation as a result of changes in mechanical properties and LIF concentration. To demonstrate that cells collected from the gels could be used for essentially any complementary downstream assay, we performed quantitative RT–PCR on selected samples. Such analyses showed how the expression of some genes associated with pluripotency was significantly downregulated (Rex1), while others (Nanog) remained largely unchanged as a result of changes in the physicochemical environment ( Fig. 4h ). Using this approach, the expression of early germ layer markers could also be assessed, and suggested that changes in 3D matrix stiffness resulted in significant upregulation of Map2 , a gene associated with early neuroectodermal differentiation. Using these techniques, it was also possible to compare self-renewal and proliferation between conventional 2D and optimized 3D culture conditions, which revealed very different colony morphologies by imaging, significantly lower proliferation in 3D as assessed by flow cytometry and notably higher expression of Nanog and Sox2 as evaluated by PCR ( Supplementary Fig. 9 ). Taken together, the possibility to perform these multimodal readouts, including time-lapse imaging, flow cytometry and PCR, opens up broad avenues for looking at cellular systems in these microarrayed 3D niches. Although 2D combinatorial material arrays, which have gained increasing popularity in recent years, have yielded invaluable insight into extrinsic stem cell regulation [28] , [29] , they cannot be expected to faithfully reproduce certain key physiological features of the in vivo microenvironment, notably spatial constraints, stiffness-mediated mechanotransduction and appropriate mode of presentation of ligands, which can only be assessed in in vitro culture by 3D cell encapsulation [13] , [30] , [31] . Although recent studies have provided initial efforts in implementing combinatorial approaches to 3D cell culture [32] , [33] , [34] , they have been limited in scope due to constraints in the ability to generate large-scale libraries of microenvironments, limited systems-level analysis and lack of cell recovery. Here, our bioengineered approaches offer new perspectives for quantitative studies in 3D and for disentangling the heterogeneity of stem cell microenvironmental components. By incorporating systems-based analysis techniques, we were able to uncover previously unknown relationships between disparate classes of elements regulating stem cell fate. We envision these tools could serve as a generic template for a more physiological and systematic approach to cancer and stem cell research. Thus, the components of interest in a target microenvironment could seamlessly be interchanged to be cell- and tissue-type specific in order to deconstruct at will specific niches found in vivo . The approach we have described here could be widely applicable by the adoption of liquid handling robots similar to the one we have used and which are available at most academic core screening facilities. In addition, the advent of increasingly widespread and inexpensive 3D printers with capabilities for dispensing biological material could allow such approaches to become even more widely accessible to individual labs. With such tools, we hope to begin understanding the role of extrinsic regulatory cues involved in morphogenesis or tumour progression across multiple levels of modulation. Hydrogel precursors synthesis Branched PEG-vinylsulphone (PEG-VS) was produced and characterized as described elsewhere [29] . Briefly, 8-arm 40-kDa PEG-OH (NOF Corporation, Japan) in dichloromethane was reacted with 100-fold molar excess over OH groups of divinylsulphone (Sigma-Aldrich, Switzerland) and filtered, washed and precipitated in diethyl ether. The final product was dried under vacuum and stored under argon at −20 °C. In a second step, PEG-VS was functionalized with FXIIIa-peptide substrates via Michael-type addition. We have used a glutamine-containing peptide (NQEQVSPL-ERCG-NH 2 ) and different types of lysine-containing peptides with various MMP-sensitive sequences: AcFKGG- GPQGIWGQ -ERCG-NH 2 (peptide W), AcFKGG- GDQGIAGF -ERCG-NH 2 (peptide A), AcFKGG- PQGIAGQ -ERCG-NH 2 (peptide G) and AcFKGG- VPMSMRGG -ERCG-NH 2 (peptide V). Consequently, we obtained one glutamine-PEG precursor (Q-PEG) and four different lysine-PEG precursors: W-PEG, A-PEG, V-PEG and G-PEG. Functionalization and characterization of these precursors was performed as described elsewhere [11] . In brief, peptides were added to PEG-VS in a 1.2-fold molar excess over VS groups in 0.3 M triethanolamine (pH 8.0) at 37 °C for 2 h, followed by dialysis (Snake Skin, MWCO 10 k, Pierce) against ultrapure water for 4 days at 4 °C. After dialysis, the salt-free products (Q-PEG, W-PEG, A-PEG, V-PEG and G-PEG) were lyophilized to obtain a white powder. Bulk hydrogel preparation Factor XIII was reconstituted in water and activated with thrombin as previously described [11] . In brief, 1 ml of FXIII (200 U ml −1 ), Fibrogammin P1250 (CSL Behring) was activated in the presence of 2.5 mM CaCl 2 with 100 μl of thrombin (20 U ml −1 , Sigma-Aldrich) for 30 min at 37 °C. Aliquots of activated factor XIIIa were stored at −80 °C for further use. Precursor solutions to give hydrogels with a final dry mass content ranging from 1.5 to 4% were prepared by stoichiometrically balanced ([Lys]/[Gln]=1) solutions of Q-PEG and each of the four lysine-PEGs in Tris buffer (50 mM, pH 7.6) containing 50 mM CaCl 2 . The cross-linking reaction was initiated by 10 U ml −1 thrombin-activated factor XIIIa and vigorous mixing. To obtain disc-shaped matrices, the liquid reaction mixtures (50 μl) were sandwiched between sterile hydrophobic glass microscopy slides (obtained by treatment with SigmaCote, Sigma) separated by spacers ( ca . 1 mm thickness) and clamped with binder clips. The matrices were then incubated for 30 min at 37 °C. MMP degradability characterization Three 50 μl gel disks at 3.5% w/v PEG were made for each of the four peptide sequences and allowed to swell for 12 h in 50 mM Tris, 100 mM NaCl, 10 mM CaCl 2 buffer at pH 7.5. They were then weighted and placed in a 40 nM MMP-1 solution (LubioScience), dissolved in the same buffer. Gel mass was recorded at 2-h intervals for the first 12 h, then at t =18, 24, 48 and 72 h. Time to complete degradation was determined either directly or by linear regression (for G peptide) and inverted to give a measure of degradability. Mechanical properties characterization Gel disks ( n =3 for each MMP sensitivity) were allowed to swell in buffer for 12 h and small strain oscillatory shear rheometry was then performed. Briefly, swollen hydrogel discs of 1–1.4 mm thickness were sandwiched between the two plates of a Bohlin CV 120 rheometer (Bohlin Instruments), and compressed to circa 80% of their original thickness to avoid slipping. Measurements were then conducted in constant strain (5%) mode. Shear stress was recorded over the frequency range of 0.1–1 Hz and average storage moduli G’ over the frequency range were obtained. Storage modulus (G′) was plotted as function of hydrogel %PEG w/v for each of the four MMP sensitivities. Linear interpolation was performed on the G′ versus %PEG data points. The % PEG corresponding to 0, 600, 1,200 and 1,800 Pa was determined for each degradability ( Supplementary Fig. 2 ). Gel tethering of cell–cell interaction proteins To tether cell–cell interaction proteins to the hydrogel network, we used an Fc-tag/Protein A conjugation strategy. To render Protein A susceptible for FXIIIa-catalysed cross-linking, we conjugated Q-containing peptide to the Protein A using NHS-PEG-maleimide, a heterobifunctional PEG linker. The modification of Protein A was achieved in a two-step reaction: functionalization with maleimide group by reaction of NHS-PEG-maleimide in tenfold molar excess, followed by Q-peptide attachment via its cysteine side chain ( Supplementary Fig. 1B ). Consequently, the (Q peptide - protein A)-functionalization was qualitatively assessed by SDS–PAGE ( Supplementary Fig. 1C ). A fluorescent counter-reactive substrate for FXIIIa, lysine-containing probe, Lys-Tamra (AnaSpec), was chosen for detecting whether FXIIIa-mediated cross-linking reaction can occur. On mixing of Protein A and Lys-Tamra in the presence of FXIIIa, a fluorescent signal corresponding to Protein A was detected on SDS–PAGE and in-gel fluorescence scanning, demonstrating successful bioconjugation. To achieve tethering of cell–cell interaction proteins into FXIIIa-based hydrogels, Fc-tagged mouse E-Cadherin, human EpCAM and human Jagged 1 (R&D Systems) were premixed with Q-Protein A in a 1.66 molar excess ratios for 30 min at room temperature. Considering that Protein A has five Fc-binding sites, we have allowed for three times molar excess of the protein of interest for each Fc-binding site, which should ensure optimal immobilization of proteins. The obtained solutions of fully functional proteinaceous constructs were aliquoted and stored at −20 °C until further use. Determination of ECM proteins susceptibility for FXIIIa We hypothesized that large-sized ECM proteins could be natural substrates for FXIIIa and would tether to the hydrogel network without further conjugation. ECM proteins of interest were purchased in solution form: mouse laminin 1, collagen IV (both mouse, BD Biosciences) and human fibronectin (human, R&D Systems). We performed a fluorescent binding assay, in which proteins were mixed with each of the fluorescent FXIIIa-substrates (Q-peptide-Alexa647 or Lys-Tamra) in the presence of FXIIIa. The reactions were qualitatively analysed by SDS–PAGE and in-gel fluorescence scanning, demonstrating that indeed the proteins are susceptible for FXIIIa-based cross-linking ( Supplementary Fig. 1C ). All ECM proteins were aliquoted at 4C and stored at −20 °C. Cell culture In all experiments (except viability assay), R1 Oct4 enhanced GFP mouse embryonic stem cells (mESC) (kindly provided by the Zandstra lab) were routinely cultured on gelatin-coated dishes in medium containing 15% serum (Hyclone) and mouse 10 3 U ml −1 LIF (ESGRO, Millipore). Twelve hours before the experiment, the medium was changed to serum-free knockout medium KnockOut TM Serum Replacement, Life Technologies. Viability assay A viability assay was carried out to compare cell behaviour in 2D and 3D conditions. Wild-type mESCs were trypsinized and seeded on a gelatin-coated tissue culture dish (2D) or encapsulated in a 600 Pa non-degradable (A) hydrogel disk (3D) at 1 million cells per ml. Incubation at 37 °C, 5% CO 2 was carried out for 4 h in +LIF serum-free conditions, followed by staining with LIVE/DEAD Cell Viability Assay (Life Technologies), following the manufacturer’s instructions. Conventional (2D) or confocal (3D) fluorescence imaging was carried out, followed by manual counting of the proportion of live (green) versus dead (red) cells carried out on three independent samples. Robotic mixing and dispensing To achieve the combinatorial complexity of this approach, we used a Hamilton Microlab StarPlus automatic liquid handling robot with Nanopipettor head ( Supplementary Fig. 4 ). All automated steps were programmed with MicroLab Vector Software version 4.1.1 (HAMILTON Bonaduz AG). Stock solutions of premixed stoichiometrically balanced PEG solutions corresponding to the four peptides were prepared by mixing glutamine-PEG precursor (Q-PEG) with the four different lysine-PEG precursors: W-PEG, A-PEG, V-PEG and G-PEG. Each of these four stock solutions was diluted to the rheology-determined four corresponding concentrations required to achieve matched target stiffnesses. The dilution and all subsequent steps of the process were performed robotically, with fluid handling parameters optimized for every material class and checked by mass measurement on a balance. Importantly, 30% of the total final volume was left empty (spare volume) to account for subsequent addition of proteins, cells and FXIIIa (10% of total volume for each component). These 16 combinations were aliquoted into 256 wells of a 384-well plate. EC and CC proteins were thawed on ice, diluted to a concentration of 500 nM and placed into the wells of a cooled 384-well plate. The four EC proteins (including blank control) were dispensed into the 256 gel precursor-filled well, followed by the four CC proteins, in an orthogonal manner such as to obtain at the end of this step 256 unique combinations of MP, DG, EC and CC (4 × 4 × 4 × 4). A 96-well plate was prepared with the mediums containing three soluble factors and a blank control: FGF4, BMP4 at 10 ng ml −1 (R&D Systems) and LIF at 10 3 U ml −1 (Millipore) final concentrations. Cells were trypsinized and resuspended in serum-free medium at a concentration of 1 × 10 6 cells per ml and kept on ice. Simultaneously, frozen aliquots of FXIIIa were thawed and also kept on ice. Next, in a sequential manner, cells were dispensed into eight wells of the mixed gel precursors, quickly followed by dispensing and robotic mixing of FXIIIa. Immediately following the addition of FXIIIa and before onset of gelation (circa 2–3 min), the 8-channel Nanopipettor was used to aspirate 12.5 μl from each well and dispense 1 μl in 12 wells of a 1,536-well plate. This process was repeated a total of 8 times per 1,536-well plate (8 channels × 8 times × 12 drops per channel per time=768 drops) to fill half of a 1,536-well plate. Throughout the process the 1,536-well plate was cooled to 4 °C to prevent evaporation. At the end of the gel dispensing round, the 4 different mediums in the 96-well plate were dispensed into the 1,536 experiment plate. The medium dispense steps were also carried out sequentially and were synchronized such that all gels were allowed to cross-link for ~30 min. Overall, the process from trypsinization to completion of the medium dispense took 2 h, and was carried out 4 times for the entire experiment (4 × 4 half-plates of 1,536 wells=3,072 wells). Indentation testing In experiments focusing on mechanical properties, a technique was developed to measure stiffness by indentation in each of the 384 wells ( Supplementary Fig. 7 ). A compression tester (TA.XT Plus Texture Analyze, Stable Micro Systems Ltd) was fitted with a custom-made 1.5-mm diameter indenting tip. Force was recorded between 0 and 70% strain. Young’s modulus was calculated from the slope of the curve between 20 and 30% strain (E low ), using the equation: where a is the radius of the indentor tip cylinder (0.75 mm), d is the indentation depth in mm, F is the recorded force in N and ν is Poisson’s ratio, taken to be 0.5. Flow cytometry and PCR analysis after gel dissociation Gels in the 384-well plate were washed with PBS for 30 min, then incubated at 37 °C with TrypLE Express (Life Technologies) cell dissociation solution for three cycles of 30 min. After each cycle, cells were collected, transferred to a round-bottom 96-well plate and kept at 4 °C. At the end of the process, wells were washed with serum-containing medium. In cases where antibody staining was carried out, SSEA-1-AlexaFluor647 (EBiosciences) at 1:100 was used according to the manufacturer’s instructions. Cells were analysed using an Accuri C6 flow cytometer (BD Biosciences). For PCR, cell dissociation was carried out with TrypleE Express as above, RNA was isolated using Tripure Isolation Reagent (Roche) according to the manufacturer’s instructions, complementary DNA was synthesized using iScript Select cDNA synthesis kit (BioRad) and RT–PCR was carried out with iQ SYBR Green Supermix (BioRad) on an Applied Biosystems 7500 machine. Imaging Imaging was carried out on a BD Pathway 435 automated imaging system (BD Biosciences). Imaging was performed on plates with live cells at D1 in the GFP channel. Plates were fixed with 4% paraformaldehyde and stained with DAPI (4',6-diamidino-2-phenylindole) at D5, followed by imaging in the GFP and DAPI channels. A × 4 objective (Olympus UPlan FLN N.A. 0.13) was used such that an entire well could be captured in a single field of view. Even at this low resolution, single cells at D1 could be distinguished. At every xy position, that is, for every well, six images were captured across a z -stack height of 800 μm. For each well, these six images in each channel were collapsed into a single additive image. The 3D information content of an entire experiment was obtained within <4 h. Image analysis All images were processed using algorithms developed in CellProfiler v.9777 (Broad Institute). For D1 analysis, collapsed image stacks for each well in the GFP channel were input. Images were thresholded and segmented. Number of cells per well was the only metric recorded for D1. All segmentations were validated by visual inspection. For D5 analysis, collapsed image stacks for each well in the GFP and DAPI channel were input. DAPI images were thresholded and segmented. Identified colony areas in DAPI were used as masks for the GFP images. For each colony, area (in pixels), average (across colony pixels) DAPI intensity and average GFP intensity were recorded. Data processing Matlab R2010b (Mathworks) was used to process and visually explore the data. Number of colonies at D1 and D5, as well as, average colony area (in pixels) and average GFP and DAPI intensity (in arbitrary fluorescence units), all at D5, were calculated by averaging single colony data for each well (3,072 data points) and for each unique condition (1,024 data points). GFP intensity was normalized to DAPI intensity, and area was converted from pixels to mm 2 . Data was further centred around the mean and rearranged by input conditions to obtain the heat maps represented in Fig. 2 . Statistical analysis Data from the 3,072 conditions was input into R V2.11. For colony area and normalized GFP intensity, GLM models, which took into account all possible interaction terms, were specified. The step Akaike Information Criterion procedure was run to obtain optimal models based on the Akaike criterion. GLM procedure of SAS v9.0 software (SAS Institute) was used to test the significance of colony area variation. Differences of LS Means±s.e.m. with the control were tested for significance. The same procedure was used to explain the variability of GFP intensity. The used models considered the effects of MP, DG, CC, EC and SF, as well as interactions determined to be significant. For all parametric tests, normality of the residues and homogeneity of the variance were examined in QQ and Tukey–Anscombe plots, respectively. Log transformations were used to improve the normality of the residues. The network interaction map, where node size was linearly proportional to the product of normalized area and normalized GFP intensity, was constructed in Cytoscape (USCD), and the interaction matrices and clustering was performed in MeV v.4.4 (TM4 Microarray Suite). How to cite this article: Ranga, A. et al . 3D niche microarrays for systems-level analyses of cell fate. Nat. Commun. 5:4324 doi: 10.1038/ncomms5324 (2014).